Second-harmonic generation using -quasi-phasematching in a GaAs whispering-gallery-mode microcavity The crystal symmetry in materials such as GaAs can enable quasi-phasematching for efficient optical frequency conversion without poling, twinning or other engineered domain inversions. symmetry means that a 90° rotation is equivalent to a crystallographic inversion. Therefore, when light circulates about the axis, as in GaAs whispering-gallery-mode microdisks, it encounters effective domain inversions that can produce quasi-phasematching. Microdisk resonators also offer resonant field enhancement, resulting in highly efficient frequency conversion in micrometre-scale volumes. These devices can be integrated in photonic circuits as compact frequency convertors, sources of radiation or entangled photons. Here we present the first experimental observation of second-harmonic generation in a whispering-gallery-mode microcavity utilizing -quasi-phasematching. We use a tapered fibre to couple into the 5-μm diameter microdisk resonator, resulting in a normalized conversion efficiency η ≈5 × 10 −5 mW −1 . Simulations indicate that when accounting for fibre-cavity scattering, the normalized conversion efficiency is η ≈3 × 10 −3 mW −1 . Frequency conversion can result from a nonlinear interaction of light with a material, where the material’s dielectric polarization responds nonlinearly with the incident electric field. Second-harmonic (SH) generation was observed in quartz more than 50 years ago [1] , [2] , when the newly developed laser was essential to observe the nonlinearlity. Efficient optical frequency conversion using these nonlinear processes requires the phases of the driving polarization and generated electric field be matched or properly compensated [3] , [4] . Consider sum-frequency generation where ω 3 = ω 1 + ω 2 (SH generation (SHG) is obtained if ω 1 = ω 2 ). For the general case of sum-frequency generation, the generated electric field at frequency ω 3 propagates as E 3 exp(- ik 3 z), while the nonlinear driving polarization propagates as χ (2) E 1 E 2 exp[− i ( k 1 + k 2 ) z ], where k i is the wavevector at frequency ω i and χ (2) is the second-order nonlinear coefficient. Perfect phasematching is achieved when k 3 = k 1 + k 2 and can be obtained by, for instance, mixing orthogonally polarized waves in a birefringent crystal [5] . Efficient conversion can also be attained using quasi-phasematching (QPM) [3] , [4] , where χ (2) is modulated at period Λ =2 πj /| k 3 − k 1 − k 2 | ( j is an integer). This modulation can be produced by periodic domain inversions where χ (2) changes sign [3] , [4] , by on-off modulation [6] , or by modulation in the magnitude of χ (2) (ref. 7 ). Materials such as GaAs that possess crystal symmetry can exhibit an effective χ (2) modulation when the fields propagate in curved geometries (such as in microrings or microdisks) [8] , [9] , [10] , [11] . A 90° rotation about the axis is the same as a crystallographic inversion, and hence fields propagating around the axis ( 001 ) in an uniform GaAs microdisk effectively encounter four domain inversions per round trip. Thus, the crystal symmetry allows QPM to be achieved without externally produced domain inversions. GaAs is particularly attractive for nonlinear frequency conversion, as it features a high nonlinear susceptibility, higher than that of LiNbO 3 and GaP [12] . Second-order nonlinear mixing has been achieved in other whispering gallery-mode resonators using other forms of phasematching. Efficient SHG has been observed in millimetre-scale disk resonators made of periodically poled LiNbO 3 (ref. 13 ) where QPM was achieved using engineered domain inversions. Birefringent phasematching was utilized to demonstrate efficient conversion in uniform LiNbO 3 disk resonators [14] , [15] . SHG was observed in a GaP photonic crystal cavity [16] . Finally, frequency conversion using four-wave mixing ( χ (3) ) has been shown in GaAs microring resonators [17] . We present here the first experimental observation of SHG in a whispering-gallery-mode resonator utilizing -quasi phasematching. The GaAs-based QPM whispering gallery-mode resonator allows for efficient SHG in micrometre-size structures that are compatible with integrated photonic architecture. These resonators could be used in all-optical circuits [18] , [19] and as integrated photonic chip sources of classical and non-classical light [20] , [21] , [22] . Basic concepts SHG in a 001 -surface-normal GaAs microdisk ( Fig. 1 ) occurs between a TE-polarized (electric field in the plane of the disk) fundamental (f) wave and a TM-polarized (electric field orthogonal to the disk plane) SH wave. These polarizations are dictated by the χ (2) tensor for GaAs and other 3 m point-group materials, which has only one non-zero susceptibility tensor element, d 14 = d xyz . 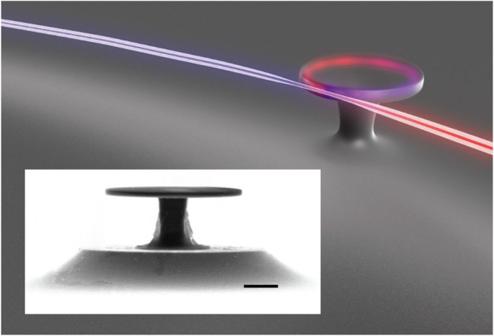Figure 1: Schematic of second-harmonic generation in a fibre-taper-coupled GaAs microdisk. Input light at the fundamental wavelength (represented by red light) is converted inside the microdisk to second-harmonic light (represented by blue light). The inset shows a scanning electron micrograph of a fabricated device. The scale bar is 1 μm. Writing the electric fields at ω i as , where i =f or SH, A i ( θ ) is the slowly varying amplitude and m i is the azimuthal number; the change in the SH amplitude with propagation angle θ is (refs 8 , 11 ) Figure 1: Schematic of second-harmonic generation in a fibre-taper-coupled GaAs microdisk. Input light at the fundamental wavelength (represented by red light) is converted inside the microdisk to second-harmonic light (represented by blue light). The inset shows a scanning electron micrograph of a fabricated device. The scale bar is 1 μm. Full size image K + and K − are the SHG coefficients calculated from mode-overlap integrals [11] (see Supplementary Discussion ) and Δ m = m SH –2 m f . Equation (1) may be integrated to obtain the increase in SH amplitude per round trip where sinc( x )=sin( x )/ x , and we have assumed A f ≈ constant. SHG is largest when the QPM condition is satisfied: Δ m =+2 or −2. This condition is equivalent to requiring that the microdisk circumference be approximately 4 π /| k SH –2 k f | [9] , [10] . Optimizing conversion with off-resonance waves While the fundamental wavelength must equal twice the generated second-harmonic wavelength by energy conservation ( λ f =2 λ SH ), the microdisk resonances are not guaranteed to be properly spaced to satisfy , where are resonance wavelengths. The most efficient SHG is obtained when both the fundamental and SH waves are resonant with the microdisk ( λ f = and λ SH = ) and the -QPM condition is satisfied (Δ m =±2). However, frequency conversion can still be obtained if one of the waves is off-resonance with the microdisk ( λ f =2 λ SH , but λ f ≠ or λ SH ≠ ), which leads to partially doubly resonant or singly resonant SHG. The generated second-harmonic spectrum, as a function of the fundamental wavelength, is proportional to [11] (see Supplementary Discussion ) where ( λ f ) and ( λ f /2) are the circulating-power spectra of the microdisk cavity in the fundamental and SH wavelength ranges, and is the SH gain coefficient defined by Equation (2). When light at λ f is coupled into the microresonator, the high circulating fundamental power generates a SH wave at λ f /2 that we desire to overlap with a resonance in the ( λ f /2) spectrum. Higher quality factors can increase SHG by increasing the resonating powers but make it more difficult to achieve overlap in the ( λ f ) and ( λ f /2) spectra. The amount of SH conversion depends on the detuning of the resonances, | −2 |, compared with their linewidths. The resonance linewidths depend on the coupling ( ) and intrinsic ( ) quality factors of the microdisk. are typically fixed by fabrication, while can be varied by adjusting coupling to the microdisk. When the resonances are aligned (| −2 |=0), maximum conversion is obtained at critical coupling ( = at both wavelengths). When the resonances are not aligned (| −2 |≠0), higher SH conversion may be produced when the cavity is overcoupled ( < ) where increased coupling broadens the resonance linewidths and produces better spectral overlap, as illustrated in Fig. 2 . Using theory presented in Kuo and Solomon [11] , we calculated SH conversion, η , for different resonance detunings, | –2 |, as is varied relative to . In Fig. 2a , is varied relative to while we fix = . In addition to the peak conversion at critical coupling = , a second maximum is obtained at / <1 when the half width at half maximum of the fundamental microdisk resonance equals the detuning. 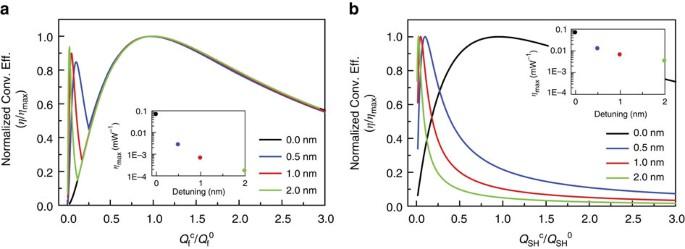Figure 2: Dependence of theoretical SH conversion efficiency on resonance detuning and quality-factor ratio. ηis normalized to its peak value and shown as a function of the ratio of coupling to intrinsic quality factors (/) for several detunings (|–2|=0, 0.5, 1.0 and 2.0 nm). It is calculated for doublingλf≈1,990 nm in a 2.6-μm-radius, 160-nm-thick GaAs microdisk where Δm=–2. The intrinsic quality factors are==20,000. Ina, critical coupling is assumed for the SH resonance (=), whileis varied relative to, while inb, critical coupling is assumed for the fundamental resonance (=) whileis varied relative to. When |–2|≠0, optimum SH conversion may be obtained by loweringand over-coupling until the half width at half maximum (HWHM) equals the detuning. The insets plot the value of maximum SH conversion efficiency (ηmax) for the different detunings. Larger detunings lead to lower conversion efficiency; however, over-coupling to broaden linewidths can improve conversion. Figure 2b shows the SH conversion when is varied relative to while we fix = . Only when | –2 |=0 is the SH conversion maximized at = . With non-zero | –2 |, the conversion efficiency is largest at lower where the SH resonance is broadened by coupling. In general, increased detunings lower the peak SH conversion (see Fig. 2 insets); however, reducing the / ratio can help mitigate the drop. Overcoupling broadens the resonance linewidths, which can lead to better spectral overlap and improved conversion. Figure 2: Dependence of theoretical SH conversion efficiency on resonance detuning and quality-factor ratio. η is normalized to its peak value and shown as a function of the ratio of coupling to intrinsic quality factors ( / ) for several detunings (| –2 |=0, 0.5, 1.0 and 2.0 nm). It is calculated for doubling λ f ≈1,990 nm in a 2.6-μm-radius, 160-nm-thick GaAs microdisk where Δ m =–2. The intrinsic quality factors are = =20,000. In a , critical coupling is assumed for the SH resonance ( = ), while is varied relative to , while in b , critical coupling is assumed for the fundamental resonance ( = ) while is varied relative to . When | –2 |≠0, optimum SH conversion may be obtained by lowering and over-coupling until the half width at half maximum (HWHM) equals the detuning. The insets plot the value of maximum SH conversion efficiency ( η max ) for the different detunings. Larger detunings lead to lower conversion efficiency; however, over-coupling to broaden linewidths can improve conversion. Full size image Frequency conversion in a GaAs microdisk cavity Experimentally, GaAs microdisks were probed using the setup sketched in Fig. 3a . Microdisk whispering-gallery-mode resonances are characterized by three integers ( m i , p i and q i ) that count the azimuthal, radial and vertical antinodes, respectively. Using a tapered optical fibre to launch and collect light from the microdisk [23] ( Fig. 3b ), we measured microdisk transmission spectra in the fundamental (1,900–2,015 nm) and SH (950–1,007 nm) wavelength ranges and identified ( m i and p i ) values of the resonances ( q f = q SH =1 for the thin microdisks used here). The resonance wavelengths and free-spectral ranges of different radial-mode families were compared with predictions from two-dimensional (2D) finite-element modelling to determine ( m i and p i ). The microdisk thickness and radius were used as fitting parameters in the modelling, and the resulting fitted sizes were consistent with observations by scanning electron microscopy (within ±5%). We characterized and (related to the total quality factor through 1/ =1/ +1/ ) by observing the changes in the transmission spectra as the gap between the fibre and microdisk was varied. The microdisks were then pumped with the fundamental beam, and the generated SH light was detected by a silicon detector. 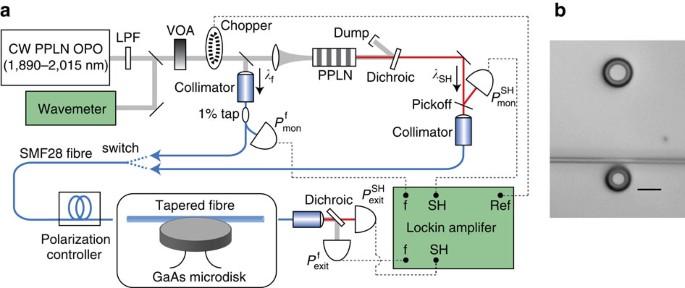Figure 3: Experimental setup. In experimental diagram (a), two fibre-coupled beams at the fundamental and SH wavelengths were produced using a continuous-wave (CW), periodically poled LiNbO3(PPLN) OPO and a PPLN doubling crystal. The beams were alternately coupled into the GaAs microdisk using a tapered fibre. The monitor (,) and exit (,) powers were recorded by a lockin amplifier. LPF, 1,850-nm long-pass filter; VOA, variable optical attenuator; dichroic filter reflects the fundamental and transmits the second harmonic. (b) Photograph of the fibre taper in close proximity to a GaAs microdisk. The scale bar is 10 μm. Figure 3: Experimental setup. In experimental diagram ( a ), two fibre-coupled beams at the fundamental and SH wavelengths were produced using a continuous-wave (CW), periodically poled LiNbO 3 (PPLN) OPO and a PPLN doubling crystal. The beams were alternately coupled into the GaAs microdisk using a tapered fibre. The monitor ( , ) and exit ( , ) powers were recorded by a lockin amplifier. LPF, 1,850-nm long-pass filter; VOA, variable optical attenuator; dichroic filter reflects the fundamental and transmits the second harmonic. ( b ) Photograph of the fibre taper in close proximity to a GaAs microdisk. The scale bar is 10 μm. Full size image We fabricated GaAs microdisks with 2.6-μm radius and 160-nm thickness using molecular-beam epitaxy, photolithography and wet chemical-etching (see Methods for details). Figures 1 (inset) show images of the GaAs microdisk cavities. All fabricated microdisks showed misaligned fundamental and SH resonances (| –2 |≠0). 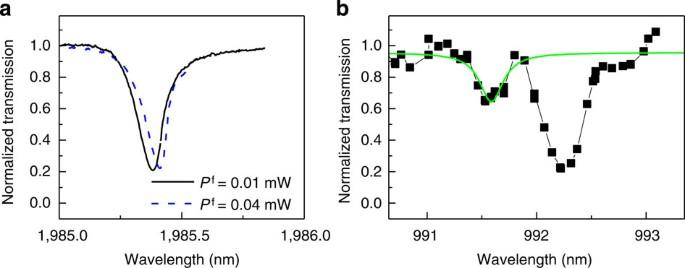Figure 4: Measured transmission spectra of the microdisk cavity. (a) TE-polarized transmission spectra of the (mf=13,pf=1) resonance near 1,985 nm at two power levels. (b) TM-polarized, transmission spectrum (black) near 990 nm along with fit (green) to the (mSH=24,pSH=2) resonance. Figure 4 plots the fundamental and SH transmission spectra for the GaAs microdisk with the smallest detuning, measured with the fibre taper contacted to the microdisk. We chose to touch the fibre to the top edge of the microdisk to increase measurement stability and increase coupling, as suggested by Fig. 2 for non-zero detuning. We identified the TE-polarized, fundamental resonance centred at 1,985.38 nm as ( m f =13, p f =1). At the SH wavelength, we observed two TM-polarized resonances in the vicinity of 992 nm. By probing these resonances with various taper-disk separations and taper sizes, we determined that the resonance at 991.6 nm is ( m SH =24, p SH =2) and the resonance at 992.25 nm is ( m SH =21, p SH =3). We also observed the ( m SH =28, p SH =1) resonance at 997 nm. Nonlinear optical mixing using the m f =13 and m SH =21 resonances does not occur since there is no phasematching (Δ m =−5) [11] , and the ( m SH =28, p SH =1) resonance is too far detuned for efficient SHG. We conclude that SHG in the microdisk involves the ( m f =13, p f =1) fundamental resonance at 1,985.38 nm and the ( m SH =24, p SH =2) SH resonance at 991.6 nm with Δ m =−2 and detuning | –2 |=2.2 nm. Figure 4: Measured transmission spectra of the microdisk cavity. ( a ) TE-polarized transmission spectra of the ( m f =13, p f =1) resonance near 1,985 nm at two power levels. ( b ) TM-polarized, transmission spectrum (black) near 990 nm along with fit (green) to the ( m SH =24, p SH =2) resonance. Full size image In Fig. 5a , we plot the observed SH conversion efficiency ( / ) as a function of the fundamental pump wavelength. and are powers inside the fibre taper adjacent to the GaAs microdisk and are calculated based on the measured taper losses and detected powers. For this microdisk with ≠2 , SH conversion is maximized when the fundamental is on-resonance while the SH is off-resonance, as seen in Fig. 5a top inset. 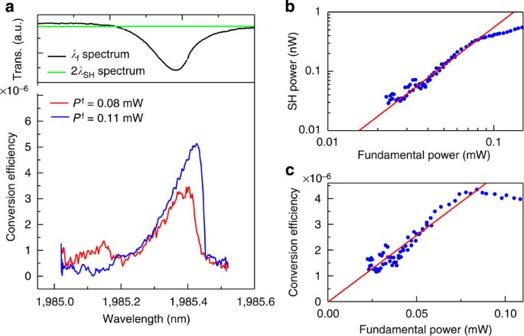Figure 5: Measure SHG spectra and dependence of SH conversion on fundamental pump power. (a) Spectrum of SH external conversion efficiency (at two fundamental powers) as a function of fundamental pump wavelength. The top inset shows the low-power resonance spectra for the fundamental and SH (in units of 2λSH) wavelengths. The spectrum in the region of the SH uses the fitting shown inFig. 4bfor themSH=24 resonance. The SH resonance is centred at 2λSH=1,983.2 nm (off-scale). (b) Logarithmic plot of generated second-harmonic versus pump power at 1,985.38-nm pump wavelength (blue dots). The fitted slope (red line) is 2.15±0.10, indicating quadratic growth of SH power with pump power. (c) SHG conversion efficiency as a function of 1,985.38-nm pump power. The slope at low power indicates (5.2±0.4) × 10−5mW−1normalized conversion efficiency; however the curve rolls off because of distortion of the resonance. Figure 5b,c plots the generated SH power and the SHG conversion efficiency in the tapered fibre, which we call the external conversion efficiency, for λ f =1,985.38 nm. At low pump power, the logarithmic plot of generated SH power ( Fig. 5b ) has a slope of 2.15±0.10, confirming quadratic growth of the second harmonic. The fitted slope at low power in Fig. 5c indicates normalized external conversion efficiency η =(5.2±0.4) × 10 −5 mW −1 . Note that this value of the conversion efficiency corresponds to absolute value and not percentage. Unless otherwise stated, this convention is assumed for all values of conversion efficiency provided hereafter. At higher pump powers, the conversion efficiency at fixed λ f rolls off primarily due to shifting of the fundamental resonance wavelength. Figure 5: Measure SHG spectra and dependence of SH conversion on fundamental pump power. ( a ) Spectrum of SH external conversion efficiency (at two fundamental powers) as a function of fundamental pump wavelength. The top inset shows the low-power resonance spectra for the fundamental and SH (in units of 2 λ SH ) wavelengths. The spectrum in the region of the SH uses the fitting shown in Fig. 4b for the m SH =24 resonance. The SH resonance is centred at 2 λ SH =1,983.2 nm (off-scale). ( b ) Logarithmic plot of generated second-harmonic versus pump power at 1,985.38-nm pump wavelength (blue dots). The fitted slope (red line) is 2.15±0.10, indicating quadratic growth of SH power with pump power. ( c ) SHG conversion efficiency as a function of 1,985.38-nm pump power. The slope at low power indicates (5.2±0.4) × 10 −5 mW −1 normalized conversion efficiency; however the curve rolls off because of distortion of the resonance. Full size image Modelling and simulations We model the conversion efficiency using two methods. We first used the semi-analytical coupled-mode theory (CMT) [11] to calculate the theoretical conversion efficiency (for further details, see the Supplementary Discussion associated with Supplementary Fig. 1 and Supplementary Table 1 ). From Fig. 4 , we observed =16,000 and =4,000. We estimated intrinsic quality factors from transmission spectra taken with the taper several hundred nanometres separated from the microdisk where 1/ ≈0, but where weak transmission dips from the modes remain, and found =33,000 and =9,000. Using these quality factors and our observed resonance detuning | –2 |=2.2 nm, the theoretical η is 1 × 10 −3 mW −1 . If the resonances of this microdisk were aligned (| –2 |=0), we expect η =8 × 10 −2 mW −1 , an 80-fold increase in conversion efficiency. By performing a series of repeated trials, we found an uncertainty of approximately ±20% in the experimental determination of and , which in turn yielded an uncertainty of ±20% in the predicted conversion efficiency. Thus, the discrepancy between the CMT predictions and the experimental results cannot be ascribed to the experimental error in the determination of the quality factors in the system. We investigated the discrepancy between the measured and CMT-derived conversion efficiencies by conducting ab initio full three-dimensional (3D) numerical simulations of the second-order nonlinear frequency-mixing process occurring in the fibre-microdisk system. These simulations are based on both 3D finite-elements-method (3D-FEM) and 3D finite-difference-time-domain (3D-FDTD) modelling (see Methods). The simulations allow us to observe the effect of the fibre lying on the microdisk cavity. There are no fitting constants or experimental parameters except for the geometry in our simulations. When excited through the fibre, the electric field distribution at the fundamental and second harmonic frequencies inside the cavity are shown in Fig. 6a,b . In addition, Fig. 6c shows the transverse nonlinear polarization distribution resulting from the second-order nonlinear interaction between the fundamental and second harmonic wavelengths, which exhibits fourfold symmetry. 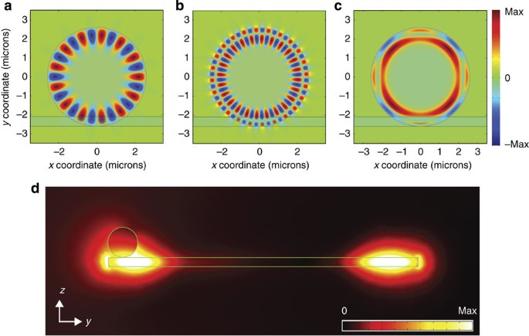Figure 6: Numerical simulations of a tapered fibre-disk system. (a) Magnetic field amplitude at the fundamental resonance evaluated in thex–yplane at the centre of the dielectric microdisk (z=0). (b) Electric field amplitude at the second-harmonic resonance evaluated in the same plane as ina. (c) Transverse polarization distribution resulting from the second-order nonlinear interaction shown ina,b. Shaded areas in the bottom region of the panels (a–c) represent the tapered fibre. Red (blue) regions in these panels indicate positive (negative) amplitudes of the corresponding field. (d) Cross-sectional view of the modulus of the fundamental electric field as computed in they-zplane atx=0. Figure 6: Numerical simulations of a tapered fibre-disk system. ( a ) Magnetic field amplitude at the fundamental resonance evaluated in the x–y plane at the centre of the dielectric microdisk ( z=0 ). ( b ) Electric field amplitude at the second-harmonic resonance evaluated in the same plane as in a . ( c ) Transverse polarization distribution resulting from the second-order nonlinear interaction shown in a , b . Shaded areas in the bottom region of the panels ( a – c ) represent the tapered fibre. Red (blue) regions in these panels indicate positive (negative) amplitudes of the corresponding field. ( d ) Cross-sectional view of the modulus of the fundamental electric field as computed in the y-z plane at x=0 . Full size image From the 3D modelling of the full fibre-microdisk cavity system, we calculated a value for the normalized conversion efficiency of η =6.78 × 10 −5 mW −1 . This value is in excellent agreement with the experimental results. The simulations show that the discrepancy between the experimental results for the full system and the predictions from our CMT is partially accounted for by our experimental configuration, where the fibre taper is in contact with the top surface of the disk. As seen in our numerical simulations, the taper perturbs the electric field in the microdisk and causes increased scattering, visible as higher electric field densities outside the disk on the left side of Fig. 6d . This effect is not accounted for by the simple CMT but is included in our full 3D simulations. Using the quality-factor values from the experiment, the amount of stored energy in the fundamental mode obtained from our full 3D simulations is ~36% smaller than the one obtained from the CMT. Our CMT may be generalized to include the above mentioned effects by, for instance, modifying the CMT transfer matrix (Supplementary Equation 11 and Supplementary Fig. 1 in the Supplementary Discussion ) to include losses. The 3D simulations show that the fraction of fundamental power coupled from the tapered fibre into the microdisk is only 0.114 because of particularly strong scattering at the fundamental wavelength. In fact, we calculate that the fraction of fundamental power in the tapered fibre that is scattered is 0.861. To calculate the fraction of second harmonic coupled to the tapered fibre, we assume reversibility with respect to in and out coupling. We find the scattered power at second harmonic is small, 0.113, a consequence of the more confined field in the taper compared with the fundamental. If we account for the scattered power, the external conversion efficiency would be 3.0 × 10 −3 mW −1 , 57.6 times larger than the measured external conversion efficiency. These simulations clearly show the effects of the taper–microdisk junction and how reducing loss from this junction can significantly improve the coupling and enhance the measured SH conversion efficiency. In addition to demonstrating -QPM, our device also shows the power of resonance enhancement in enabling efficient conversion in micrometre-scale devices. Conventional, single-pass, QPM devices have large conversion efficiencies for macroscopic length scales but have low conversion when scaled to small sizes. For example, a confocally focused [24] QPM GaAs device with d 14 =94 pmV −1 (ref. 25 ) and length equal to the microdisk circumference, 2 πR =15 μm, will have η =3 × 10 −8 mW −1 . Resonant enhancement inside the GaAs WGM microdisk resonator increases the effective interaction length and is particularly useful in the micrometre-length scales for on-chip integration. While it is important to compare the SH-normalized conversion efficiency of our whispering-gallery modes shown here to other work, it is difficult to do so because, to our knowledge, this is the first result of SHG in a micrometre-scale whispering-gallery mode structure. However, some general comparisons are possible. While of millimeter size and not fabricated using planar photonic chip processing, the 3.8-mm-diameter high-Q whispering-gallery mode resonator machined in LiNbO 3 by Fürst et al. [14] has an impressive conversion efficiency of 9% with 30 μW of input power. Using semiconductor materials and photonic integrable processing, a 1.5-mm-long AlGaAs modal-phasematched waveguide and a 5-mm-long AlGaAs QPM waveguide show normalized conversion efficiencies of 7 × 10 −3 W −1 (ref. 26 ), and 0.23W −1 (ref. 27 ), respectively. Recently, Lenglé et al. [28] has provided an useful comparison of different systems. Our device of 5 μm diameter, with normalized conversion efficiency of 5 × 10 −2 W −1 (accounting for fibre-resonator scattering losses, our simulations indicate a normalized conversion efficiency of 3W −1 ) with an input power of 80 μW, compares very well. The absolute SH conversion that we observed in the GaAs microdisk is limited by thermal effects and higher-order nonlinearities. As seen in Fig. 5a , the generated SH spectrum is asymmetric even at fundamental powers as low as 80 μW. The asymmetry in the generated SH spectrum mirrors that of the transmission spectrum at the fundamental wavelength. This type of power-dependent lineshape distortion has been observed in other microphotonic devices [29] , [30] , [31] and is attributed to thermal and higher-order nonlinear effects. The lineshape distortion that limits conversion may be ameliorated by surface treatment [31] . We have for the first time experimentally observed -quasi-phasematched, SHG in a GaAs microdisk cavity. -QPM is a new QPM technique that relies on curved propagation geometries rather than engineered domain inversions. The observed normalized conversion efficiency is much higher than that of conventional, non-resonant devices scaled to comparable, micrometre sizes. Through better tuning techniques [32] , the quasi-phasematched GaAs microdisk can operate more readily in the doubly resonance regime (that is, when | –2 |=0) rather than singly resonant SHG, yielding a significant increase in the internal conversion efficiency. More efficient and robust coupling [33] , similar to that produced in other microresonator systems, will also result in increased output coupling and better integration. GaAs microdisk frequency convertors can be attractive, on-chip sources for infrared radiation and sensing, for squeezed light [22] , or for the production of entangled photon pairs [20] , [21] . New methods of sensing may be possible because of the integrated nature of infrared generation and the resonator cavity; the presence of absorbing species affects the resonance conditions and, in turn, frequency conversion in the microdisk. From a more fundamental perspective, the experimental observations reported in this work pave the way for a number of novel research avenues based on exploring the unique interplay among nonlinearity, -QPM and light–matter interactions at the micro- and nano-length scales. Microdisk cavity fabrication Molecular-beam epitaxy was used to make the sample, which consisted of a 160-nm-thick GaAs layer on top of a 1.5-μm-thick Al 0.75 Ga 0.25 As sacrificial layer. The lateral dimensions of the GaAs microdisk were defined with photolithography and a hydrobromic acid etch. A hydrofluoric acid etch was then used to remove most of the Al 0.75 Ga 0.25 As layer, leaving a narrow pedestal supporting the GaAs microdisk (see Fig. 1 ). The pedestal had negligible effect on the low-radial-order optical modes used in the experiment. Optical measurements The experiment setup is shown in Fig. 3a . The probe beam was produced by a continuous wave, 1,900–2,015-nm tunable, periodically poled LiNbO 3 optical parametric oscillator (OPO) (Lockheed Martin Aculight Argos), whose linewidth was <1 MHz. A long-pass filter blocked any leakage pump light from the OPO. To measure the resonances of the GaAs microdisks in the SH-wavelength range, a portion of the OPO light was doubled to the range of 950–1,007 nm in an oven-mounted periodically poled LiNbO 3 crystal and then sent through a dichroic filter to reject the residual OPO light. The fundamental and SH beams were launched into two separate optical fibres, which were alternately connected to the fibre taper that addressed the GaAs microdisks. The powers of both beams were monitored using a 1% fibre tap coupler for the fundamental-wavelength beam and an uncoated BK7 pickoff plate placed near Brewster’s angle for the SH-wavelength beam. A fibre polarization controller was placed immediately before the fibre taper to control the polarization of the light at the microdisk. Light in the 1,900–2,015-nm range was detected using an extended-range InGaAs detector. Light in the 950–1,007-nm range was detected by a Si detector preceded by dichroic mirror that strongly reflected any 1,900–2,015-nm light (to avoid possible two-photon absorption by the Si detector). All detected signals were sent to lock-in amplifiers referenced to a chopper at 205 Hz, and the lock-in signal amplitudes were calibrated to an optical power metre. The OPO wavelength was constantly monitored by a wavemeter. The fibre taper and microdisk samples were mounted on two separate three-axis stages and imaged using a 50 × microscope objective connected to a silicon camera. The temperature of the microdisks was stabilized at 31 °C using a Peltier heater. The taper was fabricated by pulling a SMF28 fibre using motion-controlled stages while heating with a hydrogen–oxygen torch. The taper diameter was ~500 nm, where the fibre is single mode at both the fundamental and SH wavelengths with observed transmissions of 45% and 65%, respectively. The uncertainties in fitted slopes were calculated using the 95% confidence interval analysis. Resonance identification To identify the (m i ,p i ,q i ) values of the resonances, transmission spectra of the microdisks were measured over extended wavelength ranges in the fundamental and SH bands. The 160-nm-thick GaAs microdisks only supported the lowest order vertical modes ( q f = q SH = 1 ). Transverse electric (TE) and transverse magnetic (TM) resonances were observed in the SH wavelength range, while only the TE modes were supported at the fundamental wavelength. Different radial mode families were identified by their common lineshapes and spectral separations. Finite-element method numerical modelling was used to match the resonance locations by slightly numerically adjusting the microdisk size. We also varied the taper diameter during measurements in order to change the taper-microdisk phasematching conditions, which helped us to order and identify the radial mode families. We observed series of transmission spectra as the taper approached and finally touched the microdisk, which allowed estimation of the intrinsic and coupling quality factors for the microdisk. Numerical simulations Our 3D simulations are based on the following three-step numerical approach. First, the electromagnetic response of the considered tapered fibre–disk system at the fundamental frequency was simulated by launching a HE11 waveguide mode along the tapered fibre. To ensure that a proper mode excitation is achieved in the fibre, the numerical solution of the corresponding 2D eigenvalue problem was directly fed into the input end of the fibre. This numerical profile was obtained by assuming that the power carried by the HE11 waveguide mode is the same as the fundamental input power used in our experiments. Second, we computed the current density that is induced inside the microdisk as a consequence of the temporal variation of the nonlinear second-order polarization. In this calculation, we assumed d 14 =94 pm V −1 (ref. 25 ) for the non-zero components of the second-order nonlinear susceptibility. By computing the work that the mentioned nonlinear current exerts against the EM resonance supported by the disk at the second-harmonic frequency, we obtained the corresponding energy built up in the system. Finally, we computed how the second-harmonic energy stored inside the disk couples back into the tapered fibre. In order to check the accuracy of our numerical results, the above numerical procedure was implemented using both a 3D FDTD approach (using the MIT-MEEP implementation) and a FEM (using the COMSOL Multiphysics package). Open space in both types of simulations was mimicked by using perfectly matched layers or/and scattering boundary conditions. The corresponding discretization grids were refined until a relative numerical error of <1% is achieved in all reported results. In both cases, the refractive index of the microdisk was modelled by considering the corresponding dispersion data available in the literature. The geometrical parameters of the microdisk were chosen so that its TM-polarized ( m SH =24, p SH =2) whispering-gallery mode is detuned by 2.2 nm with respect to two times the wavelength of the TE-polarized ( m f =13, p f =1) resonance. The refractive index of the fibre was assumed to be 1.44. No additional approximations, apart from the one introduced by the spatial discretization of the dielectric constant (inherent to any FDTD or FEM implementation), were introduced in the simulations, and no fitting parameters to experimental data were assumed in the calculations. How to cite this article: Kuo, P. S. et al. Second-harmonic generation using -quasi-phasematching in a GaAs whispering-gallery-mode microcavity. Nat. Commun. 5:3109 doi: 10.1038/ncomms4109 (2014).